A paclitaxel-loaded recombinant polypeptide nanoparticle outperforms Abraxane in multiple murine cancer models Packaging clinically relevant hydrophobic drugs into a self-assembled nanoparticle can improve their aqueous solubility, plasma half-life, tumour-specific uptake and therapeutic potential. To this end, here we conjugated paclitaxel (PTX) to recombinant chimeric polypeptides (CPs) that spontaneously self-assemble into ∼ 60 nm near-monodisperse nanoparticles that increased the systemic exposure of PTX by sevenfold compared with free drug and twofold compared with the Food and Drug Administration-approved taxane nanoformulation (Abraxane). The tumour uptake of the CP–PTX nanoparticle was fivefold greater than free drug and twofold greater than Abraxane. In a murine cancer model of human triple-negative breast cancer and prostate cancer, CP–PTX induced near-complete tumour regression after a single dose in both tumour models, whereas at the same dose, no mice treated with Abraxane survived for >80 days (breast) and 60 days (prostate), respectively. These results show that a molecularly engineered nanoparticle with precisely engineered design features outperforms Abraxane, the current gold standard for PTX delivery. Most cancer chemotherapeutics are hydrophobic small molecules; this is true of many of the cytotoxic agents that have been in clinical use for many decades [1] , as well as the next generation of ‘targeted’ therapeutics—currently entering the clinic—that are small-molecule drugs specific for molecular targets that are dysregulated in cancers [2] . The small size and poor solubility of many of these cancer drugs lead to fast renal clearance and poor bioavailability by the typical—oral or parenteral—routes of delivery, and leads to limited accumulation in tumours, and hence poor clinical outcomes. Unlocking the full therapeutic potential of hydrophobic small-molecule cancer drugs requires new and innovative drug formulation strategies that can be applied across a class of structurally diverse hydrophobic drugs to solve the recurring problem of poor solubility, sub-optimal pharmacokinetics (PK) and low bioavailability. An emerging approach is to package highly hydrophobic drugs into highly water-soluble nanoscale delivery vehicles (10–100 nm diameter), as objects within this size range accumulate within solid tumours due to the enhanced permeability and retention (EPR) effect, which results from an aberrant and leaky tumour vasculature and the lack of a poorly developed lymphatic drainage system in many solid tumours [3] , [4] . To this end, we have previously shown that conjugation of small molecules with an octanol–water distribution coefficient (logD) of >1.5 drives the self-assembly of the chimeric polypeptide (CP) into near-monodisperse sub-100-nm-diameter nanoparticles [5] , and that doxorubicin-loaded CP nanoparticles showed good efficacy in a subcutaneous (s.c.) murine colon cancer tumour model [6] . Those results, while promising, only suggested the clinical potential of this nanotechnology, as they were limited to a single, murine tumour in a s.c. model, the therapeutic index of this formulation was modest and the CP–doxorubicin nanoparticles were not compared with any clinically approved nanoscale formulations of the drug. This paper goes well beyond the preliminary in vivo efficacy results previously reported for CP–doxorubicin nanoparticles and assesses, through extensive in vivo experiments, the clinical potential of this nanotechnology. Clinical translation of any new nanoscale drug delivery platform requires that it be useful with more than one drug, and that it demonstrate efficacy in multiple tumours implanted at multiple—s.c. and preferably orthotopic—anatomical sites. We report herein the synthesis and in vivo delivery of near-monodisperse, sub-100-nm-sized nanoparticles that are composed of paclitaxel (PTX) conjugated to a recombinant CP that self-assembles into spherical nanoparticles upon drug attachment. The CP–PTX nanoparticles show potent tumour cell cytotoxicity, good PK and tumour accumulation, and low systemic toxicity. Notably, in a murine orthotopic tumour model of a human triple-negative breast cancer (TNBC) that is highly refractory to chemotherapy, a single intravenous infusion of CP–PTX nanoparticles showed significantly better tumour regression than Abraxane at the same dose of the drug. The therapeutic efficacy of the CP–PTX nanoparticles compared with Abraxane was even more pronounced in a s.c. prostate cancer model, as mice bearing prostate cancer tumours treated with Abraxane only survived ≤60 days, while 100% of the CP–PTX nanoparticle-treated mice survived for >70 days. These results show that a molecularly engineered nanoparticle with precisely engineered design features can outperform Abraxane—the current gold standard for PTX delivery—across multiple tumour models, which augurs well for its clinical translation. Choice of drug We chose PTX as the drug for several reasons. First, PTX is one of the most effective cytotoxic drugs to treat diverse solid tumours [7] , but it also provides a stringent test for any delivery system. This is because, with a logD of ∼ 4.95 (ref. 8 ), it is essentially insoluble in water. The second reason is that it allowed us to carry out a head-to-head comparison of our nanoparticle delivery system against Abraxane—a nanoparticle formulation of PTX bound to human serum albumin (HSA)—that is one of the few nanomedicines that have been approved by the Food and Drug Administration for cancer therapy [9] , [10] . Such direct comparisons of new delivery systems against the clinical gold standard formulation are urgently needed, but are rarely reported in the literature, which casts significant doubt on the clinical utility of many of the new ‘nanomedicines’ that are in the preclinical pipeline. Synthesis of the CP–PTX conjugate The CP consists of two chemically distinct segments: an elastin-like polypeptide (ELP), which is a disordered, and highly water-soluble recombinant peptide polymer [11] , fused to a short peptide segment containing eight cysteine residues that provide reactive sites for chemical conjugation of a chemotherapeutic of interest. The amino-acid sequence of the CP is shown in Fig. 1a . The CP was overexpressed from a plasmid-borne synthetic gene in Eshcherichia coli using a shaker-flask culture and purified from the sonicated bacterial lysate by inverse transition cycling (ITC), a non-chromatographic protein purification method described previously [12] . Three rounds of ITC provided a monodisperse product with a yield of >100 mg l −1 of purified protein. Matrix-assisted laser desorption/ionization time-of-flight mass spectrometry (MALDI-TOF–MS) showed that the molecular weight of the CP is 62,650 Da ( Fig. 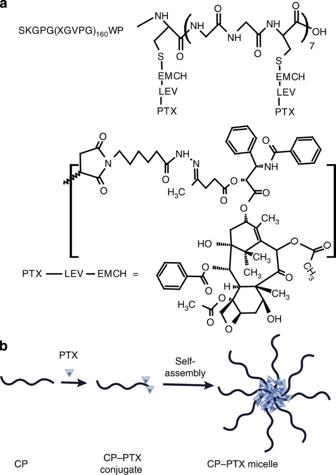Figure 1: Structure of CP–PTX conjugate and schematic of the structure of CP–PTX nanoparticles. (a) The CP was synthesized by the genetically encoded synthesis inE. coli, and conjugated to PTX at the multiple Cys residues at the C-terminal end of the CP by a pH-sensitive linker. (b) Attachment of the hydrophobic drug PTX triggers self-assembly of the CP into spherical nanoparticles with a drug-rich (blue triangles) core surrounded by a hydrophilic polypeptide corona (black chains). 2a ; Supplementary Table 1 ) and SDS–polyacrylamide gel electrophoresis (PAGE) ( Supplementary Fig. 1a ) and high-performance liquid chromatography (HPLC) confirmed that the CP had >95% purity ( Supplementary Fig. 1b ). Figure 1: Structure of CP–PTX conjugate and schematic of the structure of CP–PTX nanoparticles. ( a ) The CP was synthesized by the genetically encoded synthesis in E. coli , and conjugated to PTX at the multiple Cys residues at the C-terminal end of the CP by a pH-sensitive linker. ( b ) Attachment of the hydrophobic drug PTX triggers self-assembly of the CP into spherical nanoparticles with a drug-rich (blue triangles) core surrounded by a hydrophilic polypeptide corona (black chains). 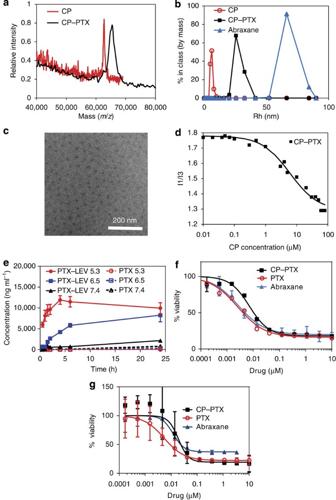Figure 2: Characterization of CP–PTX nanoparticles. (a) MALDI-MASS of CP and the CP–PTX conjugate. (b–d) Determination of hydrodynamic radius (b), cryo-TEM (c) and critical aggregation concentration (d) of the CP–PTX conjugate. (e) The kinetics of pH-dependent release of PTX from CP–PTX nanoparticles as determined by LC–MS/MS at pH 7.4, 6.5 and 5.3 (mean±s.d.). (f,g) Cell viability for CP–PTX and free PTX in MDA-MB-231 (f) and PC3 (g) cells (mean±95% CI). Full size image Figure 2: Characterization of CP–PTX nanoparticles. ( a ) MALDI-MASS of CP and the CP–PTX conjugate. ( b – d ) Determination of hydrodynamic radius ( b ), cryo-TEM ( c ) and critical aggregation concentration ( d ) of the CP–PTX conjugate. ( e ) The kinetics of pH-dependent release of PTX from CP–PTX nanoparticles as determined by LC–MS/MS at pH 7.4, 6.5 and 5.3 (mean±s.d.). ( f , g ) Cell viability for CP–PTX and free PTX in MDA-MB-231 ( f ) and PC3 ( g ) cells (mean±95% CI). Full size image To activate PTX for conjugation, it was first reacted with levulinic acid (LEV) at the 2′-OH position of PTX to introduce a keto-carbonyl functional group ( Supplementary Fig. 2 ). The product was reacted with n -ɛ-maleimidocaproic acid hydrazide (EMCH) trifluoroacetic acid to incorporate an internal, acid-labile hydrazone moiety with a terminal maleimide [6] ( Supplementary Fig. 2 ), and this activated drug was covalently attached to the Cys residues of the CP ( Fig. 1a,b ). Purified CP–PTX has ∼ 2 drug molecules per CP, as determined by MALDI-TOF–MS ( Fig. 1a ; Supplementary Fig. 3 ), as determined by the mass difference between the conjugate and the parent CP ( Supplementary Table 1 ). Characterization of the CP–PTX conjugate Upon conjugation of PTX, the CP–PTX conjugate spontaneously self-assembled into near-monodisperse spherical micelles ( Fig. 1a ). As PTX has a logD of 4.95, these results are entirely consistent with our previous observation that molecules with a logD >1.5 can trigger the self-assembly of a CP into nanoparticles [6] . To determine the molecular weight, radius of gyration ( R g ) and hydrodynamic radius ( R h ), the CP–PTX conjugate was analysed by static and dynamic light scattering (SLS and DLS). DLS of the CP–PTX conjugate in PBS at 37 °C showed nanoparticles with a R h of 32.5±0.6 nm ( Fig. 2b ; Supplementary Fig. 4b ). Analysis of the partial Zimm plot obtained from SLS showed that the R g of the CP–PTX nanoparticles was 26.6 nm and that the aggregation number of the nanoparticles was 50 ( Supplementary Fig. 4c,d ; Supplementary Table 1 ). The experimentally determined form factor ( ρ )—calculated as R g / R h —was 0.82, which is close to the theoretical value of 0.775 for spherical micelles [13] . The size and spherical morphology of the CP–PTX nanoparticles were confirmed by cryo-transmission electron microscopy (TEM), which allows for the direct visualization of self-assembled structures in a near-native, hydrated state ( Fig. 2c ; Supplementary Fig. 4g ). Only the hydrophobic core of CP–PTX nanoparticles is visualized by cryo-TEM, due to the low electron density and high degree of hydration of the ELP chains in the corona of the nanoparticles. The average nanoparticle radius determined by cryo-TEM ( R TEM , deduced from the average core-to-core distance) was measured as 23±0.4 nm ( n =50), and the average core radius ( R core ) was measured as 7.5±0.2 nm. The slight discrepancy between R TEM and the slightly larger R g and R h obtained from light scattering could be due to a slight overlap of corona chains in the vitreous ice layer or due to nanoparticle compaction during the vitrification process. We also measured the transition temperature ( T t ) of the CP–PTX nanoparticles as a function of the CP concentration in PBS ( Supplementary Fig. 4e ). The T t of the CP–PTX nanoparticles is independent of the CP concentration in the range of 25–50 μM, which is in sharp contrast to CP unimers (no PTX attached) whose transition temperatures vary significantly with their composition and concentration ( Supplementary Fig. 4e ). In PBS, the T t of the CP–PTX nanoparticles was 45 °C at 25 μM, whereas the T t of the CP ranged from 65 °C for 50 μm to 69 °C for 25 μM. We also examined the thermal response of the CP–PTX nanoparticles in 90% fetal bovine serum (a close approximation to physiological conditions). We found that the T t of CP–PTX nanoparticles decreased by ∼ 6 °C, consistent with previous results [5] ( Supplementary Fig. 4f ). Abraxane was also analysed by DLS, SLS and cryo-TEM. Light scattering showed self-assembled structures with a R g of 79 nm and a R h of 96 nm ( Supplementary Table 2 ), both of which are in agreement with the previously reported diameter of 130 nm determined by DLS [14] . The shape factor, ρ =0.83, is also close to the theoretical value of 0.775 for spherical micelles, and the aggregation number was 1,757 albumin molecules per nanoparticle, implying a highly dense structure. This high density allowed Abraxane to be visualized with high contrast by cryo-TEM, which showed that Abraxane has a somewhat irregular but approximately spherical morphology ( Supplementary Fig. 5 ). The thermodynamic stability of the CP–PTX micelles was measured by a pyrene fluorescence assay, which showed that the critical micelle concentration (CMC) of the CP–PTX nanoparticles was ∼ 1 μM ( Fig. 2d ). The CMC was confirmed by DLS as a function of CP–PTX concentration, which showed that the population with a R h of ∼ 32 nm persisted down to a concentration of 5 μM ( Supplementary Fig. 4a ), with no evidence of a second population of CP–PTX unimers. pH-dependent drug release The liberation of free drug from the CP–PTX nanoparticles requires the pH-dependent cleavage of the hydrazone and ester bond ( Fig. 1b ). To evaluate the kinetics of drug release, CP–PTX nanoparticles were incubated in buffer solutions at three different pHs: pH 7.4 (neutral), 6.5 (tumour) or 5.3 (endosomal) and at 37 °C for 24 h ( Fig. 2e ). The release of PTX–LEV and PTX was monitored by liquid chromatography–MS (LC–MS–MS). At pH 7.4, both the hydrazone and ester bond were stable, and no significant release of free drug was observed over 24 h compared with that at acidic pH. In contrast, at pH 6.5, PTX–LEV was generated at a faster rate because of cleavage of the ester bond, and reached a plateau at 24 h ( Fig. 2e ). Most strikingly, at pH 5.3, the hydrazone bond was cleaved at a much faster rate and the release of PTX reached a steady state within 8 h ( Fig. 2e ). These data confirm that the covalent conjugate of PTX is stable at the pH of blood, but that the drug is cleaved at an appreciable rate at the tumour interstitial pH (6.5) [15] and at the pH in late endosomes (pH 5.3) [16] . Hence, the pH-dependent release of PTX from the CP–PTX nanoparticle suggests slow release of the drug in the interstitial space of the tumour and a faster rate of release in the endo-lysosomal compartment following cellular uptake of CP–PTX nanoparticles. In vitro anticancer efficacy We chose MDA-MB-231, a human TNBC as the first cell line for treatment with the CP–PTX nanoparticle, because PTX is used to treat patients with TNBC [8] . TNBC is characterized by a lack of oestrogen receptor, progesterone receptor and HER-2 gene expression [17] , and 15–20% of breast cancers are triple negative [17] . Unfortunately, TNBC presents a difficult clinical challenge as it is ultimately refractory to chemotherapy [18] , and displays a shorter median time to relapse and death than other subtypes of breast cancer [18] . Treatment of MDA-MB-231 with CP–PTX nanoparticles hence provides a stringent test of the clinical utility of this nanoparticle formulation. After 72 h exposure to CP–PTX nanoparticles, the proliferation of MDA-MB-231 cells was significantly inhibited ( Fig. 2f ) and was comparable to the inhibition observed for treatment of cells with the same dose of Abraxane, and free drug in a dimethylsulphoxide (DMSO) solution diluted with PBS. Next, we evaluated the anticancer efficacy of CP–PTX in a human prostate cancer PC3 cell line. Similar to MDA-MB-231 cells, the proliferation of PC3 cells was also significantly inhibited ( Fig. 2g ) with CP–PTX treatment and that was comparable to the same dose treatment of PTX. 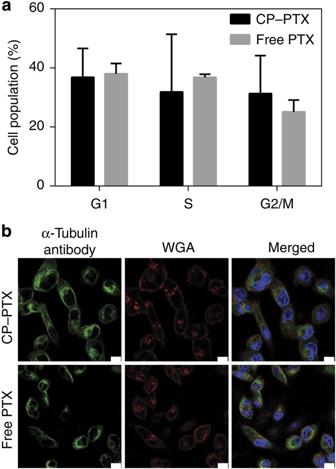Figure 3: Cell cycle arrest at the G2/M phase by CP–PTX. (a) MDA-MB-231 cells were treated with 1 nM PTX equivalent at 37 °C for 48 h. Adherent cells were collected, fixed in 70% ethanol, treated with RNase A and stained with propidium iodide (PI). Samples were analysed by flow cytometry. Results are expressed as the percentage of each subpopulation as determined by analysis of 5,000 cells per sample. (Two-way ANOVA, mean±95% CI,n=3,P<0.05). (b) Stabilization of the microtubule structure by CP–PTX in MDA-MB-231 cells. Cells were treated with 1 nM CP–PTX or free PTX at 37 °C. After 24 h, cells were stained with α-tubulin antibody (green), Hoechst 33342 (blue) and WGA (red) and imaged by confocal fluorescence microscopy. Scale bar, 10 μm. The half-maximal inhibitory concentration (IC 50 ), defined as the concentration of PTX or PTX equivalent (for the CP–PTX nanoparticles and Abraxane) needed to kill 50% of cells, was found to be 7.1 and 18.9 nM for CP–PTX, 2.5 and 5.3 nM for PTX and 2.7 and 11.9 nM for Abraxane for MDA-MB-231 and PC3 cells, respectively ( Supplementary Table 3 ). The data clearly show that the CP–PTX nanoparticles inhibit the in vitro proliferation of both MDA-MB-231 and PC3 cells, and that conjugation of PTX to the CP does not markedly decrease the activity of the drug. Stabilization of microtubule structure To investigate the mechanism by which CP–PTX inhibits cell proliferation, we examined the ability of CP–PTX to stabilize microtubules and their dynamic assembly, given that PTX’s mode of action is disruption of microtubule dynamics [19] . To do so, we quantified the population of MDA-MB-231 cells in different stages of the cell cycle upon treatment with CP–PTX or PTX at a concentration of 1 nM PTX equivalent. We chose this concentration because most cells are alive at this concentration, as we wanted to avoid the complication introduced in the analysis if a subpopulation of cells were to die during the experiment. The percentages of cell population in each phase of the cell cycle are indicated in the histograms ( Fig. 3a ). Exposure of 1 nM CP–PTX showed significant G2/M arrest (31.3 %, P <0.05 versus free drug), whereas cells treated with 1 nM of PTX had 25.1% ( P <0.05) of G2/M population ( Fig. 3a ). Figure 3: Cell cycle arrest at the G2/M phase by CP–PTX. ( a ) MDA-MB-231 cells were treated with 1 nM PTX equivalent at 37 °C for 48 h. Adherent cells were collected, fixed in 70% ethanol, treated with RNase A and stained with propidium iodide (PI). Samples were analysed by flow cytometry. Results are expressed as the percentage of each subpopulation as determined by analysis of 5,000 cells per sample. (Two-way ANOVA, mean±95% CI, n =3, P <0.05). ( b ) Stabilization of the microtubule structure by CP–PTX in MDA-MB-231 cells. Cells were treated with 1 nM CP–PTX or free PTX at 37 °C. After 24 h, cells were stained with α-tubulin antibody (green), Hoechst 33342 (blue) and WGA (red) and imaged by confocal fluorescence microscopy. Scale bar, 10 μm. Full size image We next performed immunofluorescence studies to visualize the stabilization of microtubules by cells treated with CP–PTX. MDA-MB-231 cells were stained with an α-tubulin antibody 48 h after treatment with CP–PTX or free PTX to visualize microtubules, and cell nuclei were stained with Hoechst 33342. After 48 h exposure of CP–PTX and PTX to MDA-MB-231 cells, the multipolar spindles were replaced by microtubule bundles and the nuclei were dumbbell shaped in both CP–PTX and free PTX-treated cells ( Fig. 3b ). Determination of PK of the CP–PTX conjugate To evaluate and compare the plasma half-life, the CP–PTX nanoparticles, Abraxane and free drug were administered systemically and the plasma drug concentration was measured as a function of time post injection ( Fig. 4a ). The free drug was administered as the clinical parenteral formulation, consisting of PTX dissolved in a mixture of Cremophor EL (polyoxyethylated castor oil) and ethanol (50:50, v/v), which is diluted right before injection [20] . 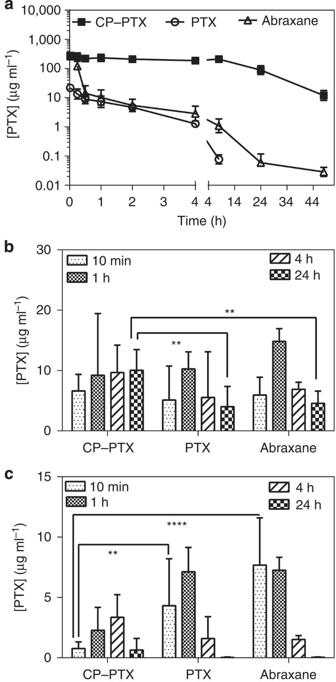Figure 4: Plasma pharmacokinetics and tissue biodistribution. (a) Plasma PTX concentration as a function of time post injection. A non-compartment model was fitted to the plasma PTX concentration, which yielded a terminal half-life of 8.4 h for CP–PTX and 3.8 h for Abraxane (mean±95% CI,n=4). (b,c) The PTX concentration in tumour (b) and muscle (c) at 10 min and 24 h post administration of free PTX, Abraxane and CP–PTX nanoparticles.**P<0.01 and****P<0.0001 (two-way ANOVA, Tukey’s test; mean±95% CI,n=4). Figure 4: Plasma pharmacokinetics and tissue biodistribution. ( a ) Plasma PTX concentration as a function of time post injection. A non-compartment model was fitted to the plasma PTX concentration, which yielded a terminal half-life of 8.4 h for CP–PTX and 3.8 h for Abraxane (mean±95% CI, n =4). ( b , c ) The PTX concentration in tumour ( b ) and muscle ( c ) at 10 min and 24 h post administration of free PTX, Abraxane and CP–PTX nanoparticles. ** P <0.01 and **** P <0.0001 (two-way ANOVA, Tukey’s test; mean±95% CI, n =4). Full size image The measurement of PTX concentration and the various PTX degradation products for the CP–PTX nanoparticles is non-trivial because PTX is not fluorescent, and radioactively labelling PTX is both tedious and expensive. We employed LC–MS–MS analysis to determine the in vivo concentration of PTX for free drug, Abraxane and the various CP–PTX products liberated from the nanoparticles by acid cleavage. The pharmacokinetic parameters were calculated using a non-compartment pharmacokinetic approach within WinNonlin software ( Supplementary Information ), yielding a terminal half-life for the CP–PTX nanoparticles of 8.4±1.9 h and a plasma area under the curve (AUC) of 5,135±447 μg ml −1 h ( Supplementary Table 4 ). In contrast, the terminal half-life for mice treated with the same dose of free PTX and Abraxane are only 1.2±0.4 h ( Supplementary Table 4 ) and 3.8±0.7 h ( Fig. 4a ; Supplementary Table 4 ) and the AUC of free PTX and Abraxane are 27.0±8.1 μg ml −1 h and 80.8±45.1 μg ml −1 h, respectively. As PTX is linked to LEV through an ester bond, and the PTX–LEV conjugate is in turn conjugated with EMCH through a hydrazone bond in the CP–PTX conjugate, CP–PTX can potentially release PTX and PTX–LEV over time in systemic circulation. Hence, we also measured the AUC and terminal t 1/2 for both PTX and the PTX–LEV conjugate. The AUCs for PTX and PTX–LEV in mice treated with the CP–PTX nanoparticles are 15.6±2.2 μg ml −1 h and 125.4±16.0 μg ml −1 h, respectively, while the terminal t 1/2 of PTX and PTX–LEV are 13.5±10 h and 10.7±2.8 h, respectively ( Supplementary Table 4 ). These results clearly show that the CP–PTX nanoparticles provide a sevenfold-higher plasma exposure than free drug and more than twofold-higher plasma exposure than Abraxane, which is a necessary pre-requisite for enhanced accumulation in solid tumours via the enhanced EPR effect [4] . We next evaluated the in vivo biodistribution of PTX delivered to tumours by systemically injected CP–PTX nanoparticles and Abraxane. Mice were administered free drug as the Cremophor formulation, Abraxane or CP–PTX nanoparticles, and tissue samples of treated mice were collected after 10 min, 1, 4 and 24 h ( Fig. 4b,c ; Supplementary Fig. 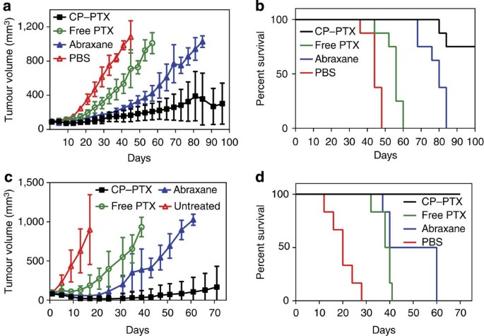Figure 5: Anti-tumour activity of CP–PTX nanoparticles. (a,b) Tumour cells (MDA-MB-231) were implanted in the mammary fat pad on day 0. When the tumour volume reached∼100 mm3, mice were treated at the MTD with PBS (n=8), free PTX (25 mg kg−1BW,n=8), Abraxane or CP–PTX (50 mg PTX equiv per kilogram BW,n=8). (a) Tumour volume up to day 100 (mean±95% CI,n=8).P=0.0001 for CP–PTX versus PTX and PBS (day 44), respectively (Tukey test). (b) Cumulative survival of mice (Kaplan Meier). (c,d) Tumour cells (PC3) were implanted on the right flank on day 0. When the tumour volume reached 50–100 mm3, mice were treated at the MTD with PBS (n=6), free PTX (25 mg kg−1BW,n=6), Abraxane or CP–PTX (50 mg PTX equiv per kilogram BW,n=6). (c) Tumour volume up to day 70 (mean±95% CI,n=6).P=0.0001 for CP–PTX versus PTX (day 30) (Tukey test). (d) Cumulative survival of mice (Kaplan–Meier). 8 ; Supplementary Table 5 ). Notably, 24 h after administration, CP–PTX showed a 2.5-fold increase in drug concentration in the tumour, as compared with free drug at the same dose ( Fig. 4b ; two-way analysis of variance (ANOVA) and Tukey’s test; P =0.01). Equally important, the CP–PTX nanoparticles significantly reduced the drug concentration at other sites in the body, including the muscle, liver, lung, kidney and heart ( Supplementary Fig. 8 ). In particular, the level of PTX delivered by CP–PTX nanoparticles in the muscle, liver, lung, kidney and heart was lower by 5.7-, 7-, 2.6-, 5.5- and 5.4-fold, respectively, compared with free PTX (two-way ANOVA and Tukey’s test; P =<0.001, <0.0001, <0.01, <0.0001, <0.01) and 9.9-, 10.7-, 27.3-, 5.3- and 4.1-fold, respectively, compared with Abraxane (two-way ANOVA and Tukey’s test; P =<0.0001, <0.0001, <0.01, <0.0001). Most importantly, following CP–PTX treatment, the concentration of PTX remains constant over time ( Fig. 4b ), whereas for free drug and Abraxane treatment, the PTX concentration decreased with time ( Fig. 4b ). The decreased accumulation in the muscle is notable, as neurotoxicity is the dose-limiting side effect of free PTX [21] . Furthermore, the accumulation of PTX in the liver is also significantly lower for CP–PTX nanoparticle-treated mice compared with Abraxane and free PTX treatments. This is important because nanoparticles typically show significant accumulation in the liver [22] , [23] . In vivo anticancer efficacy To compare the therapeutic effect of CP–PTX nanoparticles versus free PTX, both formulations were administered in a dose escalation study to determine their maximum tolerated dose (MTD). The MTD of PTX was 25 mg kg −1 body weight (BW), and the MTD for CP–PTX was ≥50 mg PTX equiv. per kilogram BW ( Supplementary Fig. 6 ). We believe that the true MTD of CP–PTX nanoparticles is >50 mg kg −1 , but we were unable to increase the dose beyond 50 mg kg −1 because of the viscosity of the solution. In any event, by administration of the CP–PTX nanoparticles at 50 mg kg −1 , it is potentially possible to increase the absolute concentration of the drug in the tumour at 24 h by an estimated fivefold over free drug while minimizing toxic side effects. The increase in tumour exposure and the decrease in exposure of the drug to muscle, liver, lung, kidney and heart is one mechanism that may explain why the MTD of CP–PTX nanoparticles is greater than that of free PTX ( Fig. 4b,c ; Supplementary Fig. 8 ; Supplementary Table 5 ), and suggested that CP–PTX nanoparticle formulation may improve the therapeutic index of PTX. CP–PTX nanoparticles were first evaluated for their in vivo anti-tumour activity in a s.c. MDA-MB-231 xenograft model ( Supplementary Fig. 7 ) with a dose of 30 mg kg −1 BW to compare with the anti-tumour efficacy of PTX at a similar dose. Significant tumour regression with improved survival was observed in mice treated with CP–PTX compared with PTX ( Supplementary Fig. 7 ). Next, we evaluated the tumour regression efficacy of CP–PTX in an orthotopic MDA-MB-231 model. Mice with MDA-MB-231 tumours were treated once intravenously with PBS, PTX at its MTD (25 mg kg −1 ), CP–PTX nanoparticles at 50 mg kg −1 of PTX equivalent and Abraxane, also at 50 mg kg −1 of PTX equivalent ( Fig. 5a ). At 6 weeks after treatment, CP–PTX-treated mice had a mean tumour volume of 150 mm 3 ( n =8) versus 216 mm 3 ( n =8) for Abraxane, 535 mm 3 ( n =8) for free drug- (Tukey’s test; P =0.0001) and 985 mm 3 ( n =8) for PBS-treated controls (Tukey’s test; P =0.0001). Clearly, the CP–PTX formulation outperforms Abraxane and free drug in reducing tumour volume, which correlated with a substantial increase in animal survival ( Fig. 5b ). This is notable as free PTX was ineffective in controlling tumour growth. The median survival time for mice treated with PBS ( n =8) was 44 days, and treatment with the Cremophor formulation of PTX ( n =8) slightly increased this survival to 56 days (Kaplan–Meier, Wilcoxon test, P <0.0001). Treatment with Abraxane further increased the survival to 80 days (Kaplan–Meier, Wilcoxon test, P <0.0001). In contrast, six out of eight mice were alive for up to 100 days after treatment of CP–PTX nanoparticles, and two of eight mice had no residual tumours ( Fig. 5b ). These results clearly demonstrate that treatment with CP–PTX significantly improved the survival of mice bearing orthotopic MDA-MB-231 tumour over free drug (Kaplan–Meier, Wilcoxon test, P <0.0001) and Abraxane (Kaplan–Meier, Wilcoxon test, P <0.0001). Figure 5: Anti-tumour activity of CP–PTX nanoparticles. ( a , b ) Tumour cells (MDA-MB-231) were implanted in the mammary fat pad on day 0. When the tumour volume reached ∼ 100 mm 3 , mice were treated at the MTD with PBS ( n =8), free PTX (25 mg kg −1 BW, n =8), Abraxane or CP–PTX (50 mg PTX equiv per kilogram BW, n =8). ( a ) Tumour volume up to day 100 (mean±95% CI, n =8). P =0.0001 for CP–PTX versus PTX and PBS (day 44), respectively (Tukey test). ( b ) Cumulative survival of mice (Kaplan Meier). ( c , d ) Tumour cells (PC3) were implanted on the right flank on day 0. When the tumour volume reached 50–100 mm 3 , mice were treated at the MTD with PBS ( n =6), free PTX (25 mg kg −1 BW, n =6), Abraxane or CP–PTX (50 mg PTX equiv per kilogram BW, n =6). ( c ) Tumour volume up to day 70 (mean±95% CI, n =6). P =0.0001 for CP–PTX versus PTX (day 30) (Tukey test). ( d ) Cumulative survival of mice (Kaplan–Meier). Full size image To rule out any possibility that the ELP carrier could itself potentiate an anti-tumour effect, we intravenously injected ELP (1,900 mg kg −1 ELP) or co-injected ELP (1,900 mg kg −1 ELP) and PTX (25 mg kg −1 ) in mice bearing orthotopic MDA-MB-231 tumours. The ELP treatment had no effect on tumour growth or animal survival, and was similar to tumour growth and survival of PBS-treated mice. Furthermore, mice co-treated with ELP and PTX had a virtually identical response as mice treated with PTX ( Supplementary Fig. 13 ). These results clearly confirm that the ELP has no direct cytotoxicity. To investigate whether these results would translate across tumour types, we next selected PC3, a human prostate tumour, as a second tumour target. PC3 xenografts were implanted s.c. in male nude mice and were treated with a single dose of PTX (25 mg kg −1 ), CP–PTX nanoparticles or Abraxane (both at 50 mg kg −1 ). Mice treated with CP–PTX nanoparticles had a mean tumour volume of 23 mm 3 ( n =6) versus 216 mm 3 ( n =6) for Abraxane (Tukey’s test; P <0.01) and 549 mm 3 ( n =6) for free drug (Tukey’s test; P <0.05) 30 days after treatment. Clearly, the CP–PTX formulation at the MTD vastly outperforms Abraxane and free drug in reducing tumour volume, which correlated with a substantial increase in animal survival ( Fig. 5b ). This is notable as free PTX is totally ineffective in controlling tumour growth. The median survival time for mice treated with PBS ( n =8) was 20 days, and treatment with PTX ( n =8) slightly increased survival to 39 days (Kaplan–Meier, log-rank test, P <0.0001). Treatment of Abraxane further increased survival to 50 days (Kaplan–Meier, log-rank test, P <0.0001). In contrast, all six mice were alive for up to 70 days after treatment of CP–PTX nanoparticles ( Fig. 5b ). Thus, with only a single-dose injection, CP–PTX nanoparticles provide a substantial curative effect. Gene expression analysis of tumours To explore the mechanism by which CP–PTX nanoparticles outperform the free drug, we next compared the genomic profiles for tumours obtained from mice treated with PBS, free PTX and CP–PTX. To determine the change in gene expression profile change over time, we also compared the genomic profiles of the response phase and relapse phase for both CP–PTX and free PTX-treated tumours. Global gene expression analysis clearly showed that the gene expression profile of the CP–PTX response samples was distinct from all the other four remaining groups of samples (untreated control, PTX response, PTX relapse and CP–PTX relapse), and these differences were even larger than the differences between the controls versus treated samples ( Supplementary Data 1 ). To determine the effect of the empty vehicles on the gene expression of xenografts, global gene expression of the ELP-treated tumour was compared with that of PBS treatment. These experiments showed that ELP treatment had a minimal effect on the gene expression profile of xenografts ( Supplementary Fig. 14 ). To define the changes of each probe set associated with each treatment, we performed a zero transformation against the average expression levels of the same probe sets of the control tumours, as described previously [24] , [25] . At least a twofold change of 1,647 probe sets was found between groups and that was arranged by hierarchical clustering according to similarities in expression patterns ( Fig. 6a ). This analysis highlights the distinct gene expression changes associated with the CP–PTX-treated tumours with several clusters of genes that were only repressed or induced in the CP–PTX samples ( Fig. 6a,b ). For example, CP–PTX-treated tumour showed significant repression of a large cluster of genes that are involved in DNA proliferation and repair, such as BubR1 , centrosome components ( CENPF and CENPE ), PCNA and PARP1 . In addition, several genes involved in fibrosis were also repressed in the CP–PTX-treated tumour, including lysyl oxidase (LOX) and fibronectin (FN1). In contrast, a large cluster of genes were induced only in the PTX response, PTX relapse and CP–PTX relapse samples, but not in the CP–PTX response samples. This cluster contains the adhesion molecule CD24 and several genes that are known to be induced by hypoxia, including LOX , PGK1 , BMIP3L and VEGFC . 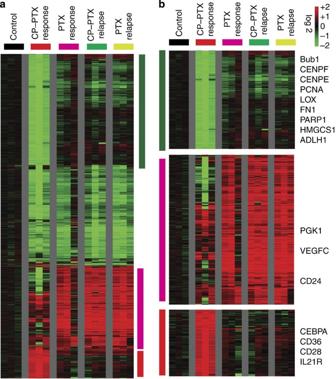Figure 6: Gene expression analysis of tumours treated with CP–PTX or PTX. (a) The global gene expression of xenografts that are responsive to treatment with CP–PTX nanoparticle or PTX or relapse upon treatment was determined using microarray analysis using U133A2 (Affymetrix) arrays. The transcriptional response of each treatment was derived by zero transformation. Selected gene clusters, which were induced and repressed specifically in the CP–PTX tumours, that responded to treatment are highlighted by the colour bar. (b) The three gene clusters that reflected the distinct changes in the CP–PTX response tumours were further expanded with selected names shown. Figure 6: Gene expression analysis of tumours treated with CP–PTX or PTX. ( a ) The global gene expression of xenografts that are responsive to treatment with CP–PTX nanoparticle or PTX or relapse upon treatment was determined using microarray analysis using U133A2 (Affymetrix) arrays. The transcriptional response of each treatment was derived by zero transformation. Selected gene clusters, which were induced and repressed specifically in the CP–PTX tumours, that responded to treatment are highlighted by the colour bar. ( b ) The three gene clusters that reflected the distinct changes in the CP–PTX response tumours were further expanded with selected names shown. Full size image To identify the underlying biological processes that are affected by treatment with CP–PTX nanoparticles, we used gene set enrichment analysis [26] —a method to identify the enrichment or depletion biological processes as represented by gene sets—to perform pairwise comparison between CP–PTX response and the untreated control, CP–PTX relapse and the untreated control as well as CP–PTX response and CP–PTX relapse. The most enriched and depleted pathways are presented in Supplementary Data 1 . We found that the response to CP–PTX treatment, but not the CP–PTX relapse samples, was associated with the depletion of the transforming growth factor beta (TGF-β) pathway (TGF-β pathway and SMAD2) and branched-chain amino-acid catabolism ( Supplementary Fig. 15 ). The tumours’ response to CP–PTX nanoparticle treatment was also associated with the enrichment of genes in the classical adipogenic target of PPAR-γ, immune gene clusters and sensitivity to chemotherapies and γ-radiation. From the microarray data, we also studied some oncogenic pathways of the tumours treated with either CP–PTX or PTX. These data show the upregulation of genes related to interferon gamma (IFNγ), IFNα and downregulation of E2F1, PI3K, EFGR, hypoxia, and genes involved in TGF-β signalling ( Supplementary Fig. 16 ). While taxanes are highly effective drugs for many cancers, the toxicity associated with solubilization strategies [27] , [28] and the side effects that arise from nonspecific drug accumulation in healthy organs provide motivation for the development of better delivery technologies. A liposomal formulation of PTX improved solubility of the drug and showed similar in vitro cytotoxicity against a variety of tumour cell lines compared with the Cremophor formulaiton (Taxol) [29] , but in vivo results of this formulation in a solid tumour were, however, not reported. In an alternative approach, taxanes have been physically encapsulated in synthetic polymer micelles (for example, Genexol [30] and NK105 (ref. 31 )). However, in most cases, physically encapsulated taxanes are rapidly released from polymeric micelles and bind with serum proteins, so that the improvement in plasma half-life over the Cremophor formulation only leads to a modest improvement in efficacy over free drug [30] , [32] , [33] . Abraxane—a ∼ 130-nm-diameter particle of PTX physically bound to HSA—is the most promising, and the only clinically approved nanoparticle carrier of PTX at this time, as it shows greater efficacy in preclinical models than the Cremophor formulation of PTX and lower systemic toxicity in human patients [23] , [34] , [35] , [36] , [37] , [38] . An alternative approach to physical encapsulation is the covalent conjugation of the drug to a synthetic polymer. XYOTAX, a polyglutamic acid–PTX conjugate showed promising preclinical results, but the typical taxane side effects of hypersensitivity, neuropathy and neutropenia have been observed in Phase Ia and Ib clinical trials [39] . Another issue with XYOTAX is that the polyglutamate chain is hydrolytically labile, leading to rapid production of small polymer fragments of PTX during systemic circulation and nonspecific biodistribution with high uptake in the kidneys, heart and reticuloendothelial system (RES)—liver and spleen—organs [36] . The plasma elimination half-life of Abraxane and XYOTAX (polymeric conjugate) have been measured as 6.2 h (Abraxane) and 5.3 h (XYOTAX), respectively [22] , [33] , [40] . In our hand, Abraxane, despite being a nanoparticle formulation, had an elimination half-life only of 3.8±0.7 h, which is similar to other polymeric formulations of PTX. The lower plasma half-life of PTX in mice treated with Abraxane as compared with the 9.5-h -long half-life of HSA in mice [41] suggests that the drug does not remain associated with the protein long enough to fully leverage the favourable PK of HSA. This is consistent with a report that Abraxane does not exhibit tumour-selective distribution of PTX that might be expected from a long circulating drug that can take advantage of the EPR effect, as it exhibits significant and promiscuous deposition in the prostate, liver, seminal vesicles, lung, pancreas, spleen, gastrointestinal tract and kidney in a rat model [22] . In contrast, the accumulation of CP–PTX—and PTX released from CP–PTX nanoparticles—is significantly lower (2.6–27-fold) in the muscle, liver, heart, kidney and lung compared with the Abraxane and free drug. Global gene expression analysis of tumour tissue suggests that treatment with CP–PTX nanoparticles leads to the inhibition of genes such as TGF-β , E2F1 , epidermal growth factor receptor ( EGFR ) and hypoxia, which are related to tumour cell proliferation, immune surveillance, survival and poor prognosis. Importantly, upregulation of IFNγ and the interleukin-21 receptor-related gene can potentially increases the cytolytic function of macrophages, natural killer cells and cytotoxic T lymphocytes. Significant repression of a large cluster of genes that are involved in DNA proliferation and repair, such as BubR1 , centrosome components ( CENPF and CENPE ), PCNA and PARP1 , was also observed in a global gene expression analysis of tumour tissue and is consistent with a recent report that mitotic arrest alone is not responsible for the in vivo efficacy of PTX, but is related to chromosome missegregation on highly abnormal, multipolar spindles, which contributes to the in vivo efficacy of PTX, in addition to mitotic arrest [42] . Collectively, these results suggest that treatment with CP–PTX nanoparticles has a markedly different effect on gene expression within the tumour than treatment with free drug. These striking differences in the gene expression profiles, combined with similar observations for CP–doxorubicin nanoparticles [6] , suggest that the effect of a nanoparticle drug is not identical to that of the free drug at the molecular level. Whether this is simply because of differences in the rate and amount of accumulation of the drug within different subcellular compartments of cells within tumours or whether it reflects a more fundamental redefinition of the pharmacology of the drug at the molecular level is an unanswered question, and one that we will pursue in future studies. Beyond its efficacy, the CP–PTX nanoparticle formulation has several other useful attributes that augurs well for its translation to the clinic. First, synthetic polymeric micelles and polymer conjugates are more complicated to synthesize than the genetically encoded polypeptide described herein. Many synthetic polymeric vehicles are also not biodegradable, nor have they been shown to self-assemble across a broad range of hydrophobic molecules. In contrast, the CP nanoparticle system is a simple and rationally designed recombinant polypeptide that is extraordinarily efficient to synthesize and purify from E. coli , is biodegradable [43] , [44] and self-assembles into nearly monodisperse sub-100-nm nanoparticles in water upon conjugation of hydrophobic drugs, thereby obviating the need for complex processing of the drug and carrier. Attachment of hydrophobic drugs solely at the chain end ensures that the drug is sequestered in the nanoparticle core, unlike other nanoparticle drug carriers, such as dendrimers [3] , metal nanoparticles [45] or carbon nanotubes [46] that expose the hydrophobic drugs at the nanoparticle–water interface. Similar to other polypeptide– and protein–drug conjugates [47] , the attachment of the drug through an acid-labile bond limits its premature release in systemic circulation and promotes release of the drug in regions of acidic pH, such as in the acidic extracellular space of solid tumours [48] and within cells, thereby limiting spillover of the drug into circulation and healthy tissues. We believe that this combination of features makes CP nanoparticles attractive for the delivery of the many hydrophobic chemotherapeutics that are clinically approved and other drug candidates that are abandoned along the clinical pipeline because of their unfavourable physicochemical properties and poor bioavailability. Synthesis of CPs The ELP segment of the CP used for conjugation to PTX consists of the sequence SKGPG-(XGVPG) 160 -WPC(GGC) 7 (single amino-acid codes) where the guest residue X=V:G:A in a 1:7:8 ratio. Expression and purification of CP The ELP was expressed from a pET-24b expression plasmid and transformed into an E. coli strain BL21(DE3) using a previously published hyperexpression protocol, which relies on the leakiness of the T7 promoter [49] . Fifty microlitres of cultures grown for 16 h were used to inoculate six 1-l flasks of TB DRY supplemented with 45 μg ml −1 kanamycin. Each 1-l flask was then incubated at 37 °C and 210 r.p.m. for 24 h, after which the cell suspension was centrifuged at 3,000 r.p.m. for 10 min at 4 °C. Each ELP was purified using ITC, which has been described elsewhere [12] . Briefly, the cell pellet was resuspended in PBS and lysed via sonication on ice for 3 min (10 s on, 40 s off) (Masonix S-4000; Farmingdale, NY). Polyethyleneimine 0.7% w/v was added to the lysate to precipitate nucleic acid contaminants. The supernatant was then subjected to multiple rounds of ITC as follows. The solution was heated to 37 °C in the presence of 3 M NaCl. The coacervate was centrifuged for 10 min at 14,000 g and 20 °C, and resuspended in 20 mM Tris(2-carboxyethyl)phosphine hydrochloride (TCEP) in water, pH 7. This suspension was cooled to 4 °C, and then centrifuged for 10 min at 14,000 g and 4 °C to remove any insoluble contaminants. Typically, three rounds of ITC generated a sufficiently pure product (>95% by SDS–PAGE). Purity analysis Following CP purification, SDS–PAGE was performed on Bio-Rad ReadyGels with a 4–20% Tris gradient. The gels were visualized by copper staining (0.5 M CuCl 2 ). HPLC was also used to determine the purity of CP and the CP–PTX conjugate, using a LC10 HPLC (Shimadzu Scientific Instruments; Columbia, MD). For HPLC analysis of the CP, a Shodex OHPak KB-804 column (New York, NY) and an isocratic flow of 1.0 ml min −1 of water:acetonitrile:formic acid (70:30:0.05) was used. For HPLC analysis of the CP–PTX conjugate, a Shodex OHPak SB-804 column and an isocratic flow of 0.5 ml min −1 of PBS:acetonitrile (70:30) was used. The HPLC data were quantified by the integrated area under the peak at an absorbance of 228 nm, corresponding to the absorbance of PTX. Synthesis of the CP–PTX conjugate Synthesis of the PTX–LEV conjugate . PTX–LEV was synthesized as described previously [50] . Briefly, LEV (0.08 g, 0.7 mmol) and N , N ′-dicyclohexylcarbodiimide (0.145 g, 0.7 mmol) were dissolved in dry dimethylformamide (DMF), mixed with each other and stirred for 30 min at −20 °C. PTX (0.5 g, 0.58 mmol) and 4-dimethylaminopyridine (0.5 g, 0.58 mmol) were dissolved in dry DMF and were added to the above mixture. The reaction mixture was left stirred for 24 h at 4 °C. The reaction mixture was filtered and the DMF was evaporated to dryness. The compound was purified by column chromatography with silica gel and 1.5% methanol (MeOH) in chloroform as eluent. Retention factor ( R f ): 0.48 in EtOAc/hexane=2:1. Synthesis of activated PTX (PTX–LEV–EMCH) and conjugation of PTX with CP . PTX–LEV (0.05 g, 0.05 mmol) and EMCH (0.018 g, 0.07 mmol) was dissolved in dry MeOH and left stirring in the dark for 36 h at 45 °C. Next, the MeOH was evaporated to dryness and the compound was purified by silica gel column chromatography with 2–2.5% MeOH in chloroform as the eluent. PTX–LEV–EMCH was immediately used for the next step. R f : 0.6 in 10 % MeOH in CHCl 3 . Electrospray ionization (ESI)–MS: 1,159 [M+H]. 1 H NMR (400 MHz, DMSO-d6): δ 10.24 (s, 1H, 12′), 9.28 (d, 1H, −HNBz), 7.97/7.7/7.67 (5H, aromatic: O-Bz), 7.82/7.48 (5H, aromatic: N-Bz), 7.44/7.17 (5H, aromatic: Ph3′-), 6.99 (s, 2H, 12′), 6.27 (s, 3H, 10-OCOCH 3 ), 5.97 (m, 1H, 13), 5.4 (d, 1H, 2), 5.25 (dd, 1H, 3′), 4.91 (m, 1H, 5), 4.61 (d, 2H, 2′), 4.09 (m, 1H, 7), 3.99 (dd, 2H, 4-CCH 2 O), 3.57 (m, 1H, 3), 3.37 (m, 2H, 5′), 3.33(s, 3H, 10-OCOCH 3 ), 3.17 (t, 2H, 4′), 3.16 (t, 3H, 11′), 2.6 (m, 2H, 6), 2.35 (m, 2H, 7′), 2.25 (s, 3H, 6′), 2.1 (s, 3H, 4-OCOCH 3 ), 1.82 (s, 3H, 8-CH 3 ), 1.75 (d, 2H, 14), 1.48 (s, 3H, 12-CH 3 ), 1.49 (m, 2H 8′), 1.23 (m, 2H, 10′), 0.992/1.01 (s, 3H, 15-2CH 3 s), 0.84 (m, 2H, 9′). 13 C NMR: (125 MHz, DMSO-d6): δ 207.8, 202.35, 190.22, 174.52, 171.78, 171.05, 169.59, 166.279, 165.19, 155.51, 139.41, 134.43, 131.51, 129.92, 129.55, 128.64, 128.25, 127.56, 127.42, 127.23, 83.55, 80.18, 76.61, 75.20, 74.69, 70.67, 70.36, 65.31, 57.35, 54.47, 46.02, 42.87, 36.48, 34.40, 33.49, 32.97, 31.97, 29.75, 27.79, 26.30, 25.84, 24.65, 22.38, 21.36, 20.64, 16.76, 13.92, 9.72. High-resolution MS (ESI): m / z calcd for C 62 H 71 N 4 O 18 ([M+H] + ): 1,159.476341, found: 1,159.47380. Prior to conjugation with activated PTX, purified CP was suspended in reaction buffer (0.1 M NaPO4, 1 mM EDTA, pH 7.0) and reduced with 1 ml of TCEP at neutral pH (100 mM, pH 7.0) at ∼ 5 × excess to thiol. Excess TCEP was removed from the solution by initiating the phase transition with sodium chloride (2.5 M) and centrifugation at 4,000 r.p.m. at 25 °C for 10 min. The CP pellet obtained by centrifugation was resuspended in ∼ 2 ml of reaction buffer. Purified PTX–LEV–EMCH was resuspended in ∼ 2 ml of DMF and slowly transferred to the stirring CP solution. One millilitre of pH-neutral TCEP (100 mM) was added and the reactants were stirred for 16 h at 20 °C in the dark. After reaction, the unreacted PTX–LEV–EMCH precipitate was separated by centrifugation at 13,000 r.p.m. at 10 °C for 10 min. The supernatant was further purified by diluting it in 20% acetonitrile in PBS and centrifuging the solution in an Amicon Ultra-15 Centrifugal Filter Units (MWCO: 10 kDa, Millipore) at 2,500 r.p.m. at 10 °C. The CP–PTX solution was washed twice with NH 4 HCO 3 solution (pH 7.4) and then freeze dried. Determination of PTX conjugation ratio The conjugation ratio of PTX to CP was determined by MALDI-TOF–MS of the CP–PTX conjugates and free CP using a Voyager DE-Pro MALDI-MS (Applied Biosystems) instrument equipped with a nitrogen laser (337 nm). The MALDI-TOF–MS samples were prepared in an aqueous 50% acetonitrile solution containing 0.1% trifluoroacetic acid, using a sinapinic acid matrix. The conjugation ratio was determined by examining the increase in mass of the conjugate relative to free CP. Dynamic light scattering DLS was performed to determine the hydrodynamic radius (Rh) of the CP and CP–PTX nanoparticle in the range of 5–25 μM CP concentration in the presence of 30 mM TCEP and at 25 °C using a DynaproTM plate reader (Wyatt Technology, Santa Barbara, CA), following filtration through 0.22-μm Millex-GV filters (Millipore, Billerica, MA, USA). The data were analysed with a regularization fit of the autocorrelation function, and percent intensity was converted to mass intensity using Raleigh spheres model. To obtain histograms, regularization fits were used to determine the hydrodynamic radius as weighted by the percent by mass for a random coil. SLS and DLS measurements were also performed on an ALV/CGS-3 goniometer system (Langen, Germany). Samples for the ALV/CGS-3 goniometer system were prepared in PBS and filtered through 0.22-μm Millex-GV filters into a 10-mm disposable borosilicate glass tube (Fisher). Simultaneous SLS and DLS measurements were obtained at 22 °C for angles between 30° and 150° at 5° increments, with measurements at each angle consisting of three runs for 15 s. The differential refractive index (dn/dc) was determined by measuring the refractive index at five different concentrations using an Abbemat 500 refractometer (Anton Paar, Graz, Austria). DLS data were analysed by fitting the autocorrelation function to a biexponential decay using the HDRC software package (Germany). Hydrodynamic radius was plotted against the angle and extraploted to zero. SLS data were analysed by partial Zimm plots using ALV/Dynamic and Static FIT and PLOT software to determine the radius of gyration and molecular weight. Temperature-programmed turbidimetry The transition temperature ( T t ) of each sample was calculated by recording the optical density at 350 nm as a function of temperature (1 °C per min ramp) on a temperature controlled UV–vis spectrophotometer (Cary 300 Bio; Varian Instruments, Palo Alto, CA). The T t was defined as the inflection point of the turbidity profile. All samples were analysed in PBS with CP concentrations of 25 and 50 μM, respectively. Cryogenic transmission electron microscopy Cryo-TEM was performed at Duke University’s Shared Materials Instrumentation Facility (Durham, NC). Lacey holey carbon grids (Ted Pella, Redding, CA) were glow discharged in a PELCO EasiGlow Cleaning System (Ted Pella). A 3-μl drop of a sample was deposited onto the grid, blotted for 3 s with an offset of −3 mm and vitrified in liquid ethane using the Vitrobot Mark III (FEI, Eindhoven, Netherlands). Prior to vitrification, the sample chamber was maintained at 22 °C and 100% relative humidity to prevent sample evaporation. Grids were transferred to a Gatan 626 cryoholder (Gatan, Pleasanton, CA) and imaged on a FEI Tecnai G2 Twin TEM (FEI). Determination of CMC CP–PTX was further characterized by fluorescence spectroscopy using pyrene as a probe of the local hydrophobicity, which enables measurement of the CMC of CP–PTX micelles [51] . The ratio of the first fluorescence emission peak ( I 370–373 ) and the third peak ( I 381–384 ) were plotted over a range of CP concentrations. The sigmoid of best fit was used to calculate the CMC, defined as the inflection point of the curve. pH-dependent drug release To assay for the release of drug, samples of CP–PTX (1 mg ml −1 ) were resuspended in pH 5.3 and 6.5 (with 50 mM Na 2 CO 3 ) or pH 7.4 (0.1 M NaPO 4 ) and finally diluted with acetonitrile in a volume ratio of acetonitrile:aqueous solution (0.33/1.0) (v/v). Samples were incubated at 37 °C for 0.0, 0.5, 1, 1.5, 2, 4, 6 or 24 h and quenched by dilution 1:1 (vol:vol) into pH 7.4 (0.1 M NaPO4) to return the pH to above 7.0 and thereby stop hydrolysis prior to the assay. The solution was then centrifuged at 4 °C for 1 min and stored at −80 °C. Sample preparation . Aliquots of 20 μl of the above samples were mixed with 20 μl of the deuterated paclitaxel (PTX–d5) (internal standard) and 400 μl of deionized water. After liquid–liquid extraction of analytes by 1 ml of tert-butylmethylether, the top (ether) layer was removed and solvent evaporated under a gentle stream of nitrogen. The residue was reconstituted in 100 μl of 10% acetonitrile and 0.1% formic acid in water. LC conditions . Column: Agilent, Eclipse Plus C18, 4.6 × 50 mm, 1.8 μm particle size, at 40 °C; mobile phase A: 98:2 H 2 O:acetonitrile (0.1% formic acid); mobile phase B: acetonitrile; elution gradient: 0–1 min 5–95% B, 1–2 min 95% B, 2–2.2 min 95–5% B; run time: 5 min. ESI–MS/MS conditions . Electrospray parameters (for example, declustering potential, temperature and gas flow) and mass spectrometer parameters (for example, selection of parent/daughter ions and quadrupole potential) were optimized by direct infusion of pure analytes into the ESI–LC/MS system ( Supplementary Fig. 7 ). Multiple reactions monitoring (MRM) transitions ( m / z units) monitored were as follows: PTX 854.3/285.7, PTX-d5 (internal standard) 859.3/290.7, PTX–LEV 952.5/383.6. Calibration samples in 9.72–1,200 ng ml −1 (PTX and PTX–LEV) ranges were prepared by adding known amounts of pure analytes into plasma or tissue homogenate and were analysed along with study samples. Linear response was observed in the concentration ranges measured. In vitro cytotoxicity MDA-MB-231 human TNBC cells and PC3 (PC-3M-luc-C6) human prostate cancer cells were purchased from Duke Cell Culture Facility and PerkinElmer Health Sciences, Inc., respectively, and are maintained in complete media consisting of minimum essential medium eagle (MDA-MB-231) or Gibco 11095 (PC3) supplemented with 10% fetal bovine serum, 5 mM sodium pyruvate and 5 mM non-essential amino-acid mixtures. PC3 were screened for Ectromelia, EDIM, Hantaan, LCMV, LDEV, MHV, MNV, MPV, MVM, Mycoplasma pulmonis, Mycoplasma sp., Polyoma, PVM, REO3, Sendai and TMEV GDVII. The result is negative to all pathogen mentioned above. The cell line authentication screening was done by IDEXX BioResearch using the following process: Authentication process . Cell Check 9 multiplex PCR analysis using primers specific for mouse, rat, human, African green monkey and Chinese hamster genomic DNA allows confirmation of the species of origin of a given cell line and enables as little as 1–5% inter-species DNA contamination to be detected. PC3 cell lines were also genetically authenticated using microsatellite marker (STR) analysis, which also allows intra-species contamination to be detected. The PC3 reference profile was used to authenticate the PC-3M-luc-C6 line. Cells were maintained at 37 °C and 5% CO 2 and passaged every 3 days. In vitro cytotoxicity was determined by a colorimetric assay, as follows. MDA-MB-231cells or PC3 cells (1–5 × 10 3 ) were seeded per 100 μl media on BD Falcon 96-well cell culture plates (BD; Franklin Lakes, NJ) and allowed to adhere for 16–18 h. The cell media was then removed and replaced with 100 μl complete media containing PTX, Abraxane, CP–PTX nanoparticles and incubated at 37 °C for 72 h. The plates were then removed and 20 μl of CellTiter 96 AQueous (Promega, Madison, WI) 3-(4,5,-dimethyl2-yl)-5-(3-carboxymethoxyphenyl)-2-(4-sulfophenyl)-2H-tetrazolium (MTS) reagent was added to each well. Following incubation for 2 h, the absorbance of the solution was measured at 490 nm with a Victor3 microplate reader (PerkinElmer, Waltham, MA). To calculate the IC 50 , the data were fit to the equation: viability=1/(1+(CP–PTX/IC50) p ), where CP–PTX is the effective PTX concentration in the well, the IC 50 is a measure of the dose needed to kill 50% of the cell population and p represents the slope of the sigmoidal curve. Cell cycle analysis Cells grown in six-well plates for 24 h were treated with 1 nM free PTX or drug equivalent of CP–PTX for 24 h at 37°C. The drug was then removed by aspiration of the liquid, and replaced with drug-free media. Cells were cultured for another 24 h, and both floating and adherent cells were collected. Adherent cells were collected by trypsinization. For cell cycle analysis, the cell pellet was washed with cold PBS and fixed with 300 μl cold 70% ethanol for 20 min. After fixation, the cells were collected by centrifugation, washed with PBS and resuspended in 350 μl PBS. Cells were treated with 10 mg ml −1 of RNase A (Sigma, St Louis, MO) for 30 min and then with 200 μg ml −1 of propidium iodide (PI) (Biolegend, CA) for 30 min. PI fluorescence was measured by a BD FACSCanto II flow cytometer and analysed by FlowJo software (Beckman Coulter, Fullerton, CA). A plot of forward scatter versus PI intensity was used to eliminate cell debris and cell aggregates from the analysis. Fluorescence was measured for a sample of 5,000–10,000 cells, and histograms of cell number versus PI intensity were used to determine the percentage of cells in each phase of the cell cycle. Immunofluorescence microscopy MDA-MB-231 cells were seeded at 2 × 10 4 cells per well on an eight-well coverglass slide (Electron Microscopy Sciences, Hatfield, PA). After 24 h, cells were treated with 1 nM PTX, or an equivalent concentration of CP–PTX for 1 h at 37 °C or 42 °C. The compounds were removed and cells were grown in complete media at 37 °C for 24 or 72 h. Cells were rinsed with PBS and fixed with PBS+4% paraformaldehyde. Following permeabilization with PBS+0.1% Triton X-100, cells were blocked with PBS+1% goat serum+0.5% Tween 80 for 30 min at room temperature under humidified condition. Cells were stained with a 1:50 dilution of mouse anti-α-tubulin-FITC antibody (Millipore) for 1 h at room temperature. After washing thrice with PBS, the media was replaced with Hank’s balanced salt solution containing 5 μg ml −1 Alexa Fluor 594 wheat agglutinin and 2 μM Hoechst 33342 (Invitrogen, Grand Island, NY) to stain the cell membrane and nuclei, respectively. After 10 min, cells were washed thrice with PBS before the addition of Hank’s balanced salt solution. The cells were imaged immediately on a Leica SP5 confocal microscope, using a × 63-water immersion objective. Prior to in vivo implantation, cells were resuspended twice in minimum essential media (51200-038; Invitrogen, Carlsbad, CA). MDA-MB-231 cells were administered either in the right flank or mammary fat pad of female nude mice by s.c. injection of 6 × 10 6 cells in a 50-μl volume for s.c. and orthotropic tumours. For the PC3 tumour model, 2 × 10 6 cells in a 50-μl volume were injected subcutaneously on the right flank of male nude mice. All animals were treated in accordance with National Institute of Health Guide for the Care and Use of Laboratory Animals under protocols approved by the Duke University Institutional Animal Care and Use Committee. Dose escalation and tumour regression MDA-MB-231 tumour model . Female nude mice (6–8 weeks old) bearing s.c. or orthotopic MDA-MB-231 tumours were treated when the mice had a tumour volume of 75–100 mm 3 . Controls or drugs were administered by the tail vein infusion (50 μl min −1 ) of 500 μl. Dose escalation was performed with free drug and CP–PTX at 5, 10, 15, 20, 25 and 30 mg kg −1 BW and 5, 10, 15, 20 and 25 mg kg −1 BW, respectively. For the s.c. MDA-MB-231 model, mice were treated with 25 mg kg −1 BW free PTX or 30 mg kg −1 BW CP–PTX and for orthotopic tumours; mice were treated with either 25 mg kg −1 BW free PTX, 50 mg kg −1 BW CP–PTX, 1.5 mM ELP (equivalent dose of ELP compared with 50 mg kg −1 BW CP–PTX) or 50 mg kg −1 BW Abraxane. PC3 tumour model . Male nude mice (6–8 weeks old) bearing s.c. PC3 tumours were treated when the mice had a tumour volume of 75–100 mm 3 . Controls or drugs were administered by the tail vein infusion (50 μl min −1 ) of 500 μl. Mice were treated with either 25 mg kg −1 BW free PTX or 50 mg kg −1 BW CP–PTX or 50 mg kg −1 BW Abraxane. Tumour dimensions and BW were measured 3–4 times a week, and the tumour volume was calculated according to volume (mm 3 )=length × width × width × 1/2. Mice were monitored for BW loss and euthanized upon exceeding 15% loss in BW or if their tumours grew to a volume >1,000 mm 3 . The MTD was determined in mice with tumours. Cumulative survival curves were compared using Kaplan–Meier analysis and the Sidak test, Tukey test, Wilcoxon test were performed using GraphPad Prism 6 software. Pharmacokinetics and biodistribution To measure PK, CP–PTX and Abraxane were intravenously infused into female nude mice (20 mg Dox equiv. per kilogram BW) via the tail vein. A blood sample (20 μl) was collected from the tail vein at 1, 15 and 30 min, and at 1, 2, 4, 8, 24 and 48 h after infusion and diluted into PBS with heparin (1,000 U ml −1 ). The blood was centrifuged (1,500 r.p.m., 10 min, 4 °C) and divided into two parts. Analysis of CP–PTX was accomplished by sample digestion by proteinase K (non-selective proteinase) and subsequent measurement of a digestion product, fragment 1 (Frag1). Frag1, or [PTX-LEV-EMCH-Cys-Gly-Gly] 2+ ion, was identified as the most suitable fragment after qualitative enhanced spectral mass analysis of the proteinase K-digested CP–PTX and subsequent optimization of the digestion conditions (duration and temperature). In undigested samples, PTX and PTX–LEV (product of physiological digestion of ELP–PTX) were measured in a separate analytical run. All measurements were performed on a LC/ESI/tandem MS (LC–ESI–MS/MS) instrument consisting of a Shimadzu 20A series LC system and an Applied Biosystems MDS Sciex 4000 QTrap tandem mass spectrometer with ESI (ESI–MS/MS) operated in MRM mode within Analyst v. 1.4.2 software. CP–PTX sample preparation . Aliquots of 5 μl of plasma or 30 μl of tissue homogenate (one part tissue (g)+two parts deionized water (ml) were mixed with 10 μl of the PTX-d5 (internal standard) and 50 μl of 500 μg ml −1 freshly prepared proteinase K in Tris buffer pH 7.4, incubated at 55 °C for 3 h, and then diluted with 100 μl of deionized water. Solid-phase extraction . (1) Cartridge conditioning: 2 × 1 ml MeOH+2 × 1 ml H 2 O, (2) transfer of the incubated sample into the cartridge, (3) rinsing: 2 × 1 ml H 2 O and (4) elution: 0.75 ml 100% MeOH. The solvent was evaporated and residue reconstituted in 100 μl of 10% acetonitrile and 0.1% formic acid in water. PTX, Abraxane and PTX–LEV sample preparation . Aliquots of 20 μl of plasma or tissue homogenate (one part tissue (g)+two parts water (ml); tough tissues cryo-crushed before homogenization) were mixed with 20 μl of the PTX–d5 (internal standard) and 400 μl of deionized water. After liquid–liquid extraction of analytes by 1 ml of tert-butylmethylether, the top (ether) layer was removed and the solvent evaporated under a gentle stream of nitrogen. The residue was reconstituted in 100 μl of 10% acetonitrile and 0.1% formic acid in water. LC conditions . Column: Agilent, Eclipse Plus C18, 4.6 × 50 mm, 1.8 μm particle size, at 40 °C; mobile phase A: 98:2 H 2 O:acetonitrile (0.1% formic acid); mobile phase B: acetonitrile; elution gradient: 0–1 min 5–95% B, 1–2 min 95% B, 2–2.2 min 95–5% B; run time: 5 min. ESI–MS/MS conditions . Electrospray (for example, declustering potential, temperature and gas flow) and mass spectrometer (parent/daughter ions, quadrupole potential) parameters were optimized by direct infusion of pure analytes into the ESI–LC/MS system ( Supplementary Fig. 9 ). The MRM transitions ( m / z units) monitored are as follows: PTX 854.3/285.7, PTX-d5 (internal standard) 859.3/290.7, CP–PTX (as Frag1) 695.4/523.8 and PTX–LEV 952.5/383.6. Calibration samples in 9.72–1,200 ng ml −1 (PTX and PTX–LEV—plasma), 8.75–324 ng ml −1 (PTX and PTX–LEV—tissue), 125–1,000 ng ml −1 (ELP–PTX—plasma) and 12.15–1,500 ng ml −1 (ELP–PTX—tissue) ranges were prepared by adding known amounts of pure analytes into plasma or tissue homogenate and were analysed along with study samples ( Supplementary Figs 10–12 ). Linear response was observed in the concentration ranges measured. To obtain estimates and confidence intervals of pharmacokinetic parameters describing this behaviour, the data set was fit to a two-compartment pharmacokinetic model using SAAMIITM (University of Washington, Seattle, WA). The plasma concentration ( n =4) was fit to determine the initial volume of distribution, V 0 , and t 1/2 , CL, V ss ( Supplementary Table 4 ). From these data and the dose, D , other pharmacokinetic parameters were determined including the clearance: Units, estimates and confidence intervals for the above fit are all presented in Supplementary Table 4 . To quantify PTX tissue distribution, Abraxane, free drug or CP–PTX was injected at 20 mg PTX equivalent per kilogram BW via the tail vein. At 10 min, 1, 4 and 24 h after infusion, tumour, blood and tissue samples were obtained. Blood was obtained by cardiac puncture using a heparinized needle, and plasma was isolated following centrifugation of blood (14,000 r.p.m., 10 min, 4 °C). Tissue drug concentrations were compared using two-way ANOVA, and Tukey’s test determined using GraphPad Prism 6 software. Gene expression analysis MDA-MB-231 tumour inoculation and drug administration were the same as described for the in vivo tumour regression study. When the tumour volume reached 50–75 mm 3 (for CP–PTX response and PTX response) or ∼ 200 mm 3 (for control, ELP, CP–PTX relapse and PTX relapse), orthotopic tumours were collected and immediately mixed with RNAlater reagent (Qiagen, Valencia, CA) and kept frozen at −80 °C. Total RNA was later isolated from the tumour tissues by using the RNeasy kit (Qiagen). Integrity of the RNA samples was checked by RNA electrophoresis and gel analysis with an Agilent 2100 Bioanalyzer (Agilent Technologies, Inc., Santa Clara, CA). The RNA samples were processed and probes were generated and hybridized to Affymetrix U133A arrays by the Duke University Microarray Facility according to the manufacturer’s instruction. CEL files of all samples were normalized by RMA using Expression console (Affymetrix), zero-transformed against the average expression levels of the same probe sets of the vector-expressing control HSMMs, filtered by indicated criteria, clustered with cluster 3.0 and displayed with treeview as previously described [52] . The data were then formatted for zero-transformation and gene set enrichment analysis (GSEA) using the Broad public server. All the microarray data are MIAME-compliant and have been submitted into GEO with accession number GSE3614. How to cite this article: Bhattacharyya, J. et al. A paclitaxel-loaded recombinant polypeptide nanoparticle outperforms Abraxane in multiple murine cancer models. Nat. Commun. 6:7939 doi: 10.1038/ncomms8939 (2015).